Field measurements suggest the mechanism of laser-assisted water condensation Because of the potential impact on agriculture and other key human activities, efforts have been dedicated to the local control of precipitation. The most common approach consists of dispersing small particles of dry ice, silver iodide, or other salts in the atmosphere. Here we show, using field experiments conducted under various atmospheric conditions, that laser filaments can induce water condensation and fast droplet growth up to several μm in diameter in the atmosphere as soon as the relative humidity exceeds 70%. We propose that this effect relies mainly on photochemical formation of p.p.m.-range concentrations of hygroscopic HNO 3 , allowing efficient binary HNO 3 –H 2 O condensation in the laser filaments. Thermodynamic, as well as kinetic, numerical modelling based on this scenario semiquantitatively reproduces the experimental results, suggesting that particle stabilization by HNO 3 has a substantial role in the laser-induced condensation. Owing to their impact on key human activities like agriculture, strong efforts have been dedicated in the last 70 years to seed clouds by dispersing small particles of dry ice, AgI, or other salts in the atmosphere [1] . However, the efficiency of these techniques is still debated [2] , [3] . Recently, self-guided ionized filaments [4] , [5] , [6] , [7] , [8] , generated by ultrashort laser pulses, have been proposed as an alternative approach to trigger water condensation [9] . Laser filaments are self-sustained light structures of typically 100 μm diameter and up to hundreds of meters in length, widely extending the traditional linear diffraction limit. Their formation stems from an intensity-dependent refractive index modification of the propagation medium, known as the Kerr effect, and is due to third-order nonlinear polarization of the medium. It results in self-focusing of the beam, until the intensity rises sufficiently for ionizing the air. The self-generated plasma [4] , [5] , [6] , [7] , [8] and/or negative higher order Kerr effect [10] balance the self-focusing, resulting in self-guided propagation. Filaments convey an intensity as high as 5×10 13 W cm −2 over long distances [11] , ionizing and photo-oxidising [12] the air. Both of these effects could be expected to assist water condensation. However, the Thomson process [13] , [14] , triggered by charges and typical of the Wilson chamber [15] , is irrelevant to the atmosphere because it requires supersaturation [16] , [17] . Furthermore, we recently observed that laser-induced condensation and electron densities have different behaviours as a function of the incident laser power [18] . Here, on the basis of field experiments performed under various atmospheric conditions, we show that laser filaments can induce water condensation and droplet growth up to several μm in diameter in the atmosphere as soon as the relative humidity (RH) exceeds 70%. We propose that the local photochemical formation of p.p.m.-range concentrations of hygroscopic HNO 3 substantially contributes to this effect by enabling efficient binary HNO 3 –H 2 O condensation in the laser filaments. Thermodynamic as well as kinetic numerical modelling supports this interpretation. These results offer key information to optimize the water condensation process. Laser-induced rise of particle density We investigated atmospheric water condensation initiated by the Teramobile mobile femtosecond–Terawatt laser system [19] operating continuously and generating ~10 filaments over typically 15–20 m. We shielded the latter from wind by an open chamber and sampled the aerosols alternatively at 2 cm distance from the filaments and in background atmospheric conditions. Comparing the corresponding particle densities clearly evidences the laser-induced increase of the particle number in each size class, even far below water vapour saturation ( Fig. 1a–d ). The most spectacular effect is observed on nanoparticles of ~25 nm diameter. For example, at 75% RH, the nanoparticle density typically increased by 5×10 4 –10 5 cm −3 (3–6 times the background concentration), while 10 μm particles increased by a few particles per litre (up to 30% of background). Note that these are averaged values over the volume of the protection chamber, that is, after dilution by a factor of 200–400 as compared with the active filament volume (see below). As a result, the size distribution is shifted to the larger sizes ( Fig. 1e ), evidencing the laser-induced growth of the particles. Furthermore, these particles do not re-evaporate significantly. For example, 25-nm-diameter particles have been observed to last over at least 20 min, limited by the diffusion out of the measurement chamber (see blue line in Fig. 2c ). 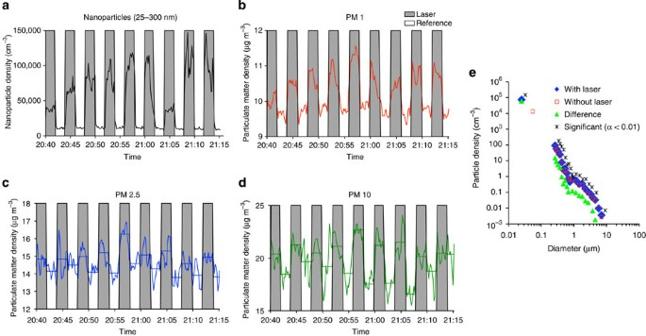Figure 1: Laser filaments-induced condensation in sub-saturated conditions. (75% RH, 13°C). (a–d) Sampling of air alternatively close to the laser (grey) and in background atmosphere. PMx denotes particulate matter of aerodynamic diameter x μm or less. On panelscandd, the average values are superimposed over the raw data. (e) Corresponding size distributions. Stars mark sizes for which a Student test yielded a statistical significance of at least 1−α >0.99 for the difference between laser and reference conditions. Figure 1: Laser filaments-induced condensation in sub-saturated conditions. (75% RH, 13°C). ( a – d ) Sampling of air alternatively close to the laser (grey) and in background atmosphere. PMx denotes particulate matter of aerodynamic diameter x μm or less. On panels c and d , the average values are superimposed over the raw data. ( e ) Corresponding size distributions. Stars mark sizes for which a Student test yielded a statistical significance of at least 1−α >0.99 for the difference between laser and reference conditions. 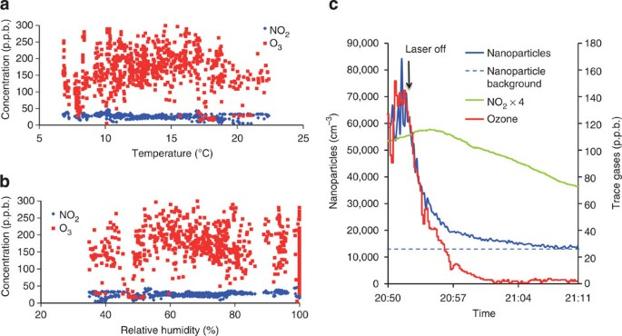Figure 2: Laser generation of trace gases. (a,b) Laser-induced concentrations of ozone and NO2as a function of (a) temperature and (b) relative humidity. (c) Temporal evolution of the concentration of nanoparticles, NO2and ozone close to the laser filaments in the protection chamber when the laser is switched off (black arrow). Nanoparticles correspond to the 25–300 nm range, with a measured median diameter close to the lower limit of 25 nm. Full size image Figure 2: Laser generation of trace gases. ( a , b ) Laser-induced concentrations of ozone and NO 2 as a function of ( a ) temperature and ( b ) relative humidity. ( c ) Temporal evolution of the concentration of nanoparticles, NO 2 and ozone close to the laser filaments in the protection chamber when the laser is switched off (black arrow). Nanoparticles correspond to the 25–300 nm range, with a measured median diameter close to the lower limit of 25 nm. Full size image Influence of atmospheric conditions Atmospheric conditions have specific and contrasted influence on the laser-assisted yield of different particle sizes. 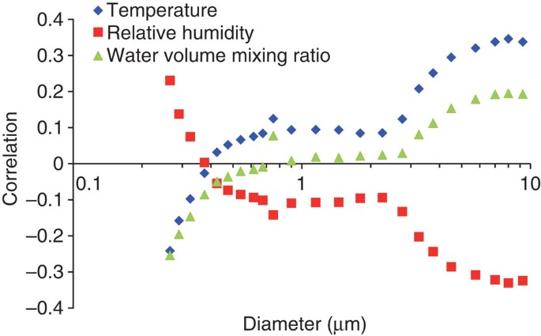Figure 3: Size-dependence of the influence of atmospheric parameters on laser-induced particles. The graph displays the correlation of temperature, relative humidity, and water mixing ratio in the atmosphere, with the laser-induced increase of particle concentration in each size class. Correlations are calculated over the whole campaign duration, each 4-minutes cycle comparing the particle concentration close to the laser filaments with that in the backgroud (Fig. 1a–d) being considered as an individual data point. As illustrated in Figure 3 , RH is positively correlated with the generation of particles below 400 nm, and negatively correlated above, whereas the opposite correlations are observed in the case of temperature. Conversely, water vapour volume mixing ratio (VMR) is anticorrelated with particles under 500 nm, positively correlated with particles above 3 μm, and uncorrelated with the generation of particles in the 600 nm–3 μm range. Figure 3: Size-dependence of the influence of atmospheric parameters on laser-induced particles. The graph displays the correlation of temperature, relative humidity, and water mixing ratio in the atmosphere, with the laser-induced increase of particle concentration in each size class. Correlations are calculated over the whole campaign duration, each 4-minutes cycle comparing the particle concentration close to the laser filaments with that in the backgroud ( Fig. 1a–d ) being considered as an individual data point. Full size image This contrasted behaviour defines three size ranges. The first one regards nanoparticles (25 nm median diameter, as compared with 55 nm in the background), the concentration of which is increased by the laser in all conditions encountered during the campaign. Their increase is positively correlated with both relative and absolute humidity ( Fig. 4b,c ), and negatively correlated with temperature ( Fig. 4a ). Particles in the 230–400 nm range feature a second regime. The effect of the laser on their concentration decreases with increasing absolute humidity ( Fig. 4f ) and temperature ( Fig. 4d ). Conversely, it is negligible below 50% RH, and increases when RH rises up to 100% ( Fig. 4e ). The dependences vanish for diameters close to 500 nm ( Fig. 4g,h,i ), and reverse above, defining the third regime ( Fig. 4j,k,l ). Note, however, that the increase of micrometer-sized particles rises again when approaching 100% RH. 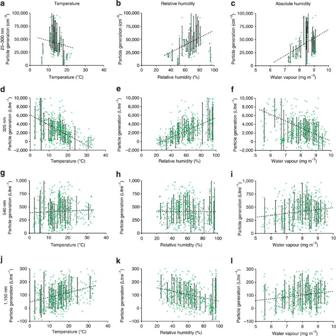Figure 4: Impact of the atmospheric conditions on laser-induced particles. Effect of laser filaments on the number density of nanoparticles (25–300 nm in diameter) (first regime, panelsa–c), 325 nm (second regime, panelsd–f), 540 nm (transition from second to third regime, panelsg–i), 1.15 μm (third regime, panelsj–l), as a function of temperature (a,d,g,j), RH (b,e,h,k), and water vapour concentration (c,f,i,l). For each size class, the difference in number density between the conditions with and without laser of each measurement cycle (Fig. 1a–d) has been considered as an individual data point, displayed as a dot on each panel of the present figure as a function of a specific atmospheric parameter. Error bars are calculated by sorting the individual measurements by increasing values of the considered atmospheric parameter, and computing one standard deviation for successive blocks encompassing 5% of the measurements. Dotted lines display linear fits of the data. Figure 4: Impact of the atmospheric conditions on laser-induced particles. Effect of laser filaments on the number density of nanoparticles (25–300 nm in diameter) (first regime, panels a – c ), 325 nm (second regime, panels d – f ), 540 nm (transition from second to third regime, panels g – i ), 1.15 μm (third regime, panels j – l ), as a function of temperature ( a , d , g , j ), RH ( b , e , h , k ), and water vapour concentration ( c , f , i , l ). For each size class, the difference in number density between the conditions with and without laser of each measurement cycle ( Fig. 1a–d ) has been considered as an individual data point, displayed as a dot on each panel of the present figure as a function of a specific atmospheric parameter. Error bars are calculated by sorting the individual measurements by increasing values of the considered atmospheric parameter, and computing one standard deviation for successive blocks encompassing 5% of the measurements. Dotted lines display linear fits of the data. Full size image Trace gas measurements Typical O 3 and NO 2 concentrations were, respectively, 200 p.p.b. and 25 p.p.b. in the open chamber, when the laser was operating, independent of the temperature and humidity ( Fig. 2a,b ). Considering the diffusion of the gases in the chamber and through its openings, the dilution factor between the filament volume and the chamber amounts to 200–400. The measured concentrations are therefore in line with laboratory results [12] , as expected resulting in a HNO 3 concentration in the p.p.m. range or above inside the filaments. Figure 2c displays the decay time of these gases, as well as of nanoparticles, after the laser is switched off. The comparable time constants for gases and particles suggests that the decay is mostly governed by dilution through the chamber apertures and owing to the airflow induced by the air sampling of the aerosol and gas sensors. The ozone concentration decreases to its background level in 10 min, faster than the nanoparticles (20 min) while NO 2 exhibits a retarded effect typical of a secondary product generated by the oxidation of NO by ozone, which also speeds up the decay of the latter. The same behaviour was observed reproducibly over more than 30 experimental realizations. 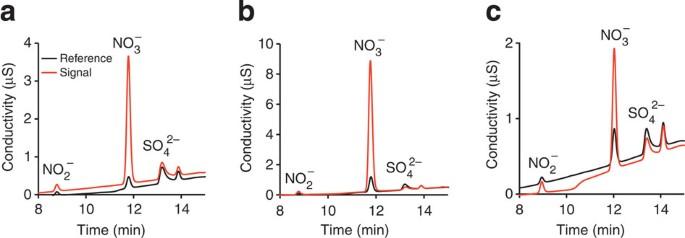Figure 5: Anionic contents of laser-induced particles. Anions are detected in the laser-induced particles by semi-quantitative ionic chromatography of particles impacted on filters with a pore of 15 nm (a), 50 nm (b) and 1 μm (c). The curves display the current detected by the chromatograph as a function of the ion transit time, characteristic of each species, for both the particles impacted on filters, and reference conditions without laser. NO 3 − contents in laser-induced particles As displayed in Figure 5 , ionic chromatography of laser-induced particles impacted on filters reveals high concentrations of HNO 3 , detected as dissolved NO 3 − ions, regardless of the particle size. This concentration is one to two orders of magnitude above that of SO 4 2− ions in the same particles. Smaller amounts of NO 2 − ions are also detected. Figure 5: Anionic contents of laser-induced particles. Anions are detected in the laser-induced particles by semi-quantitative ionic chromatography of particles impacted on filters with a pore of 15 nm ( a ), 50 nm ( b ) and 1 μm ( c ). The curves display the current detected by the chromatograph as a function of the ion transit time, characteristic of each species, for both the particles impacted on filters, and reference conditions without laser. Full size image The three different regimes observed for nanoparticles, sub-micronic, and micrometric particles suggest the following condensation mechanism. The laser initiates particle nucleation or activates pre-existing nanometer-sized particles. This nucleation from the gas phase may occur via multicomponent nucleation of sulphuric acid [20] , [21] , [22] , [23] , although it is beyond the scope of the present work in which no data is available on particles smaller than 25 nm. It results in the accumulation of ~25 nm particles inside the filaments. Such particles can grow, if the RH is sufficient to ensure their stability. Once they reach ~500 nm, their subsequent evolution is expectedly limited by diffusion of water molecules, which may explain why the growth of these particles requires high VMR, hence higher temperature, as illustrated by the correlation of both these parameters with bigger particles. On the other hand, the depletion of the humidity by the water uptake results in the negative correlation between RH and these micrometric particles. This scenario requires a highly efficient stabilizing mechanism to prevent the particles from re-evaporating well below 100% RH. This mechanism may be provided by the strong impact of the laser filaments on the local chemical composition of the atmosphere. In particular, the estimated HNO 3 concentration inside laser filaments is typically 1,000 times the p.p.b. levels at which the highly hygroscopic HNO 3 is known to stabilize water droplets in the atmosphere slightly below 100% RH (ref. 20 ). We can therefore expect efficient stabilization at much lower RH through binary HNO 3 –H 2 O condensation. The dilution factor of 200–400 between the filament active volume (~10 filaments of 100 μm typical diameter) and the protection chamber leads us to estimate that ~2×10 7 cm −3 nanoparticles, and some 10 5 cm −3 microparticles are generated in the filaments by each laser shot. Notice that up to 10 11 ozone molecules (8×10 −11 g) and 2.5×10 10 NO 2 molecules (2×10 −11 g) are available for each nanoparticle. Consequently, even larger particle sizes (several micrometers) could be stabilized by the resulting HNO 3 . These concentrations are therefore compatible with a pathway based on the binary condensation of HNO 3 –H 2 O particles. We performed numerical simulations to evaluate to what extent this binary HNO 3 –H 2 O condensation model can explain the experimental data. 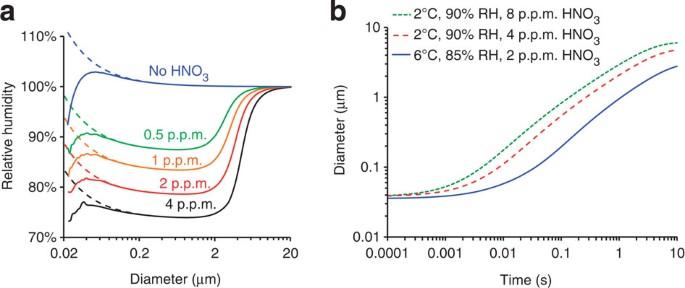Figure 6: Simulation of the droplet stability conditions and growth after the laser shot. (a) Köhler plots for a droplet density of 1,000 cm−3, at T=6°C and 1,013.25 hPa. Curves from top to bottom correspond to 0, 0.5, 1, 2, and 4 p.p.m. initial concentration of gaseous HNO3; Solid lines: Droplets including a 15 nm NH4NO3core; Dashed lines: Droplets without salt core. (b) Growth of 1,000 cm−3ternary HNO3–H2O-NH4NO3particles with a 25 nm dissolved NH4NO3core. A micrometer-sized diameter is reached within ~1 s or faster. Figure 6a displays the resulting Köhler plot, that is, the equilibrium RH over the ternary HNO 3 –H 2 O–NH 4 NO 3 droplet surface, as a function of its diameter, in conditions representative of those encountered within the laser filaments. Water-vapour uptake dominates evaporation, if the RH is higher than its equilibrium value, that is, for conditions above the curve. This value decreases down to 75% RH for a HNO 3 concentration of 4 p.p.m., allowing droplets from several tens of nm to a few μm to grow at RH well below 100% and to shift towards the right of the plot until they reach an ascending branch of the Köhler curve at several μm, consistent with the experimental data. This effect persists over the whole range of temperatures encountered in the experiment, although its effectiveness significantly decreases at rising temperatures. In particular, a higher humidity is required to stabilize the particles in warmer air. We checked that the condensation germs had no impact on the Köhler plots of particles above 80 nm, where the salt core is largely diluted (compare dotted and solid lines on Fig. 6a ), so that our results can be expected to be also representative of situations with other nucleation germs implying for example, electric charges or sulphur compounds. Figure 6: Simulation of the droplet stability conditions and growth after the laser shot. ( a ) Köhler plots for a droplet density of 1,000 cm −3 , at T=6°C and 1,013.25 hPa. Curves from top to bottom correspond to 0, 0.5, 1, 2, and 4 p.p.m. initial concentration of gaseous HNO 3 ; Solid lines: Droplets including a 15 nm NH 4 NO 3 core; Dashed lines: Droplets without salt core. ( b ) Growth of 1,000 cm −3 ternary HNO 3 –H 2 O-NH 4 NO 3 particles with a 25 nm dissolved NH 4 NO 3 core. A micrometer-sized diameter is reached within ~1 s or faster. Full size image A 15 nm salt core stabilizes the smaller particles, as shown by the positive slope of the Köhler curves for diameters below 40 nm (see solid curves on Fig. 6a ). This positive slope, which arrests the growth of the particles, constitutes a growth barrier if the RH is below the local maximum of the Köhler curve, and could therefore explain the median diameter of 25 nm observed by the nanoparticle counter, irrespective of the RH. Because RH influences the height of the Köhler maximum, and therefore the droplet capability to step over it, the Köhler plots provide a reasonable interpretation of the positive correlation between RH and the generation of particles of several hundreds of nm ( Fig. 4e ), as well as the rise of the generation of micrometer-sized particles at RH close to 100% ( Fig. 4k ). Similar results are obtained over the whole range of temperatures encountered during our campaign (2–36°C). The calculated effect of the laser decreases with increasing temperature, in agreement with the negative correlation observed in the experiments between the generation of small particles and temperature ( Fig. 4a ). The final droplet size is limited by both the amount of HNO 3 made available by the laser filaments and the water vapour VMR. Water vapour depletion occurs when the droplets exceed a few μm in diameter. This depletion is more pronounced for lower temperatures, which correspond to lower water vapour concentration for a given RH, and explains positive correlation between the concentration of larger droplets and both absolute humidity ( Fig. 4l ) and temperature ( Fig. 4j ). The laser-generated HNO 3 does not only allow the droplets to grow at a moderate relative humidity, but also drastically speeds up their growth. We reproduced this acceleration in Kulmala's model [24] in which we released the assumption of near-saturation ambient vapour pressures owing to the multi-p.p.m. HNO 3 concentration in the gas phase. As displayed on Figure 6b , in conditions representative of our experiments, the droplets typically reach a micrometer-sized diameter within ~1 s or less. Similar results have been obtained over the ranges of temperature, RH and HNO 3 concentrations representative of our experimental conditions. This fast growth is consistent with the observation of an almost instantaneous effect (on the second-scale) of the laser in the present experiments, as well as in former laboratory results [9] . In adequate conditions (see, for example, the green curve in Figure 6b ), the model even predicts a diameter increase by up to 20% within 1 ms. However, such growth is not sufficient to explain the previously observed increase of Lidar (light detection and ranging) backscattering signal only 1 ms after the filaments were shot [9] . This discrepancy illustrates the limitations of our model at the very short time scales, when the ionized and excited species within the laser-generated plasma, as well as local transient temperature jumps induced by the laser [25] strongly modify the atmospheric chemistry. Furthermore, we disregard the nucleation of new particles as well as contributions of H 2 SO 4 formed by photo-oxidation of the atmospheric SO 2 (refs 20 , 21 , 22 , 23 ), of the charges released by the filaments [26] , of mineral or organic condensation nuclei, which may be activated and made hygroscopic by the high laser-generated ozone concentrations [12] , or of other yet to be identified mechanisms. Furthermore, the information provided by the backscattering coefficient is integrated over the whole size distribution, including nanometric condensation nuclei, the formation of which is not considered in this work. Consequently, the outcome of our model cannot be directly compared with our previous size-unresolved Lidar results [9] . As a conclusion, investigations and modelling of laser-induced water vapour condensation, under various atmospheric conditions, show that laser filaments drastically increase the number density of 25 nm particles and their growth, within a few seconds, up to stable micrometric particles, even at RH as low as 70%. These nanoparticles grow in particular by condensing water vapour and HNO 3 from the atmosphere strongly modified by the laser. They form stable micrometer-sized particles that persist over at least 20 min, demonstrating that the condensation is not transient during the laser pulse, but rather a process allowing the particle growth to stable micrometer-sized droplets. Numerical modelling based on binary HNO 3 –H 2 O condensation semi-quantitatively reproduces the experimental results, although it neglects any contribution of sulphuric acid, the laser-released charges, or the activation pre-existing condensation nuclei. The simulations predict fast particle growth, their stability at low RH, and the influence of the atmospheric conditions, which confirms the substantial contribution of binary HNO 3 –H 2 O condensation in the laser filaments. Although further work is needed to characterize the nucleation of new particles, these results provide a semi-quantitative interpretation to the laser-induced condensation and define favourable atmospheric conditions for laser-assisted condensation and provide a theoretical understanding for this phenomenon. As a consequence, they open the way to applications in the real atmosphere, from remote sounding of the atmosphere to laser-based rainmaking or rain prevention. Experimental conditions Experiments were performed in 28 runs, for a total of 133 hours of records from fall 2009 to spring 2010 on the bank of the Rhône River close to Geneva (46°12' North, 6°5' East, 380 m above sea level). This location was chosen to get the benefit from the relatively warm water flow from the Lake of Geneva acting as a heat buffer, locally increasing the RH. 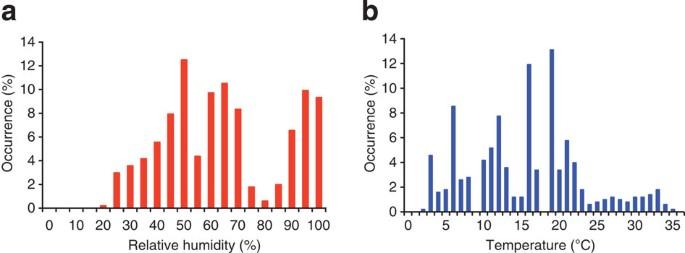Figure 7: Occurrence distribution of the atmospheric conditions during the measurements. The histograms display the statistical distribution of (a) relative humidity and (b) temperature over the whole data set acquired during the campaign, each 4-minutes measurement cycle (Fig. 1a–d) being treated as an individual datum. As detailed in Figure 7 , data were acquired in a wide variety of atmospheric conditions: RH from 35 to 100%, temperature between 2 and 36 °C. Furthermore, experiments at all times of the day and the night ensured that both phases of increase and decrease of temperature and RH have been recorded. Figure 7: Occurrence distribution of the atmospheric conditions during the measurements. The histograms display the statistical distribution of ( a ) relative humidity and ( b ) temperature over the whole data set acquired during the campaign, each 4-minutes measurement cycle ( Fig. 1a–d ) being treated as an individual datum. 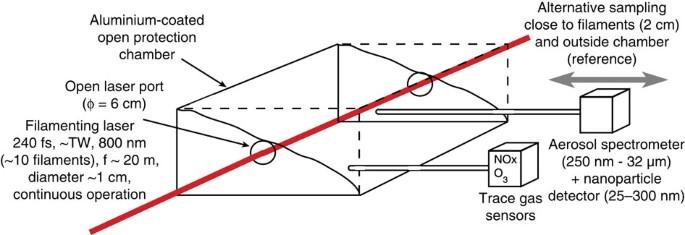Figure 8: Experimental setup. The laser filaments (red) are shielded from wind by an open protection chamber. This chamber is internally coated with aluminium and offers two widely open ports to let the laser through. Trace gases are monitored continuously in the protection chamber by dedicated sensors. The effect of the laser on aerosols is measured by sampling the particles using aerosol spectrometers and a nanoparticle detector, alternatively close to the laser filaments and in the background. Full size image Experimental setup The experimental setup is depicted schematically in Figure 8 . Water condensation was initiated by the Teramobile mobile femtosecond-Terawatt laser system [19] . The laser was operated continuously and provided up to 160 mJ pulses of 240 fs unchirped duration at a central wavelength of 800 nm and a repetition rate of 10 Hz. The beam was expanded to 10 cm diameter and slightly focused ( f ~20 m) by a built-in expanding telescope. At the nonlinear focus, that is, after ~15 m of horizontal propagation 1.2 m above ground, the beam generated some 10 filaments in the atmosphere. Filamentation spanned over typically 15–20 m, as inferred from both visual observation on a screen and the emission of a shockwave recorded by a microphone [27] . The region around the filament onset was shielded from wind by an open protection chamber (32cm×36cm×56 cm; surface-to-volume ratio 0.15 cm −1 ) where the atmosphere was analysed. This open chamber was internally coated with aluminium, and featured two circular apertures of 6 cm diameter to let the laser through. Figure 8: Experimental setup. The laser filaments (red) are shielded from wind by an open protection chamber. This chamber is internally coated with aluminium and offers two widely open ports to let the laser through. Trace gases are monitored continuously in the protection chamber by dedicated sensors. The effect of the laser on aerosols is measured by sampling the particles using aerosol spectrometers and a nanoparticle detector, alternatively close to the laser filaments and in the background. Full size image Characterization of aerosol particles After allowing typically 5 min (that is, 3,000 shots) to stabilize the aerosol and trace gas concentrations, the aerosols were sampled inside the chamber, at 2 cm distance from the filaments. Their size distribution and density were characterized using an aerosol size spectrometer (Grimm 1.107) coupled with a nanoparticle sensor (Grimm Nanocheck 1.320). The former measured the size distribution in 31 classes from 250 nm up to 32 μm based on the angular pattern of light scattering, and the latter counted and evaluated the count median diameter of nanoparticles between 25 and 300 nm by measuring the nanocurrent induced by the flow of particles after they are electrically charged in a corona discharge. Reference conditions were recorded alternatively with the laser conditions. The measurements were double-checked by intercomparing the results with other aerosol detectors. These include a second nanoparticle detector (Grimm Nanocheck 1.108), a second aerosol spectrometer (Grimm 1.107), as well as elastic optical scattering of a 1 mW continuous-wave frequency-doubled YAG laser at 532 nm. We also checked that consistent results were obtained using a condensation particle counter (TSI Model 3007), which is insensitive to the particle charge, showing that the measurement of the nanoparticles is not affected by the charges deposited on them by the filaments [28] . The statistical significance of the difference between experimental conditions was assessed by performing a Student test to calculate the risk α that the two results be due to Gaussian sampling fluctuations [29] . To ensure that the observed generation of nanoparticles is not an artefact due to the protection chamber, we performed complementary measurements without it, alternatively switching the laser on and off and sampling the aerosols at the same position. Although in this configuration we were restricted to a qualitative analysis of the data due to the perturbation by the wind airflow across the filaments, the results were consistent with the main records. We also checked that the chamber did not significantly affect the temperature and RH by performing simultaneous measurements inside and outside. We verified that the measured effect of the laser on the particle concentration is not correlated with the background particle concentrations, excluding a substantial contribution of artefacts related to the laser-induced fragmentation of pre-existing particles. The correlation between two series of values, x and y , is defined, as usual, as σ xy / σ x σ y , where σ x and σ y denote the standard deviation of the series x and y , respectively, and σ xy denotes their covariance. Substantial influence of background organic compounds was also ruled out by checking that car or ship engines running in the vicinity of our setup had minimal influence on our results; however, for safety, we disregarded the corresponding data in the analysis of our results. Chemical analysis of aerosol particles We characterized the chemical composition of the aerosols produced in the laser filaments by aspiring them at a flow of 1.2 l min −1 during 2 h of continuous laser operation and impacting them on polycarbonate membrane filters (Nuclepore Track-Etch) with 1 μm, 50 nm, or 15 nm pore sizes. Reference samples were collected without laser. Soluble particles were then dissolved by immersing the filters for 15 h in HPLC-grade water, including 15 min in an ultrasonic bath. The anions dissolved in the resulting solutions were analysed by an ionic chromatograph (ICS 3000). Trace gas measurements The influence of the atmospheric conditions on the generation of the precursors of HNO 3 , namely NO, NO 2 and ozone, was investigated by recording the gas concentrations in the protection chamber around the filament. Standard analysers monitored the concentration of O 3 , (UV Photometric Analyser Model 49, Thermo Environmental Instruments, featuring a reaction time of 20 s) as well as NO 2 , and NO (Chemiluminescent nitrogen oxides analyser AC 31 M, Environnement S.A., 15 s reaction time) in the vicinity of the filaments. Modelling of particle stability We modelled the droplet stability within the size range accessible to our experimental system, that is, above 25 nm in diameter, leaving the initial particle nucleation beyond the scope of the present work. We adapted the extended Köhler theory [30] to handle the multi-p.p.m. concentrations of HNO 3 generated by laser filaments [12] as well as the full experimental range of RH. The Köhler theory describes the equilibriums between evaporation and condensation of both water vapour and HNO 3 . It explicitly takes into account the Kelvin effect, which substantially shifts the equilibrium between evaporation and condensation because of the curvature-dependent surface energy. We neglected charge effects as well as species left in excited states in the plasma, and considered the condensational growth of a monodisperse cloud of spherical binary HNO 3 –H 2 O droplets. Within this framework, the composition- and curvature-dependent partial pressures at equilibrium are expressed as: where k B is Boltzmann's constant, T denotes the temperature, and p∞ ,i is the partial vapour pressure of species i (that is, H 2 O or HNO 3 ). The partial molecular volumes v i , the saturation partial vapour pressures p sat,i over a flat solution with the same composition as the droplet, the droplet density ρ and diameter D p , and the surface tension σ are calculated from the temperature T sol and the partial masses m i of the considered species in the liquid phase by using the thermodynamic E-AIM 'model II' ( http://www.aim.env.uea.ac.uk/aim/aim.php ) [31] , [32] , [33] . The index j denotes the dependence on all involved species. Optionally, the droplets were doped with a NH 4 NO 3 core accounting for typical nucleation germs [20] , [34] . For given salt core and water masses, we determined the equilibrium partition of HNO 3 between the gas and liquid phases, in a closed system (that is for a fixed number of HNO 3 and H 2 O molecules determined in the initial conditions). Equation (1) was then used to determine the equilibrium water vapour pressure over the corresponding droplet, defining the corresponding point in the Köhler plot. Kinetic modelling of particle growth The kinetic modelling of the droplet growth relies on the implementation of the full Kulmala's model [24] , in which we suppressed the assumption of near-saturation ambient vapour pressures owing to the low RH to handle, together with high HNO 3 concentrations in the gas phase. Mass and heat transfers between a given spherical droplet and the atmosphere are described by the classical transition regime equations [35] , including corrections for molecular diffusivities and thermal conductivity. These corrections extend the applicability of the continuum description to droplet sizes approaching the thermal molecular mean free path. Here, R is the universal gas constant, T∞ the background temperature, T a the droplet temperature, k air the thermal conductivity of air, c sol the specific heat capacity of the liquid phase. D i denotes the diffusivity of species i in air, M i its molar mass, q i its latent heat of evaporation from the mixed solution. In these expressions, heating of the atmosphere by the laser has been neglected, because it is known to keep below a few degrees [5] , [6] , [7] , [8] . f (Kn, α ) is the Fuchs-Sutugin correction factor [20] where Kn is the Knutzen number [20] (that is, the ratio of the molecular mean free path to the droplet radius). The mass and thermal accommodation coefficients α m,i and α T describe non-unity sticking probability of molecules of species i impinging the particle surface, and imperfect thermal coupling due to gas kinetic effects, respectively. We set them to unity, following the recommendation of Laaksonen et al . in the context of growth rate modelling [36] . The specific heat capacity c sol of the liquid phase is approximated by that of pure water, whereas the thermal conductivity of the atmosphere is approximated as that of pure air [35] . The effective latent heats of evaporation q i , depend on the particle composition due to the exothermic dissolution of gaseous HNO 3 . They are obtained from the equilibrium vapour pressures calculated with the E-AIM model, using the Clausius–Clapeyron equation: Using this expression neglects the distortion of the saturation vapour pressures due to the Kelvin effect, which however causes a relative change of the latent heats remaining below ~1% even for droplet diameters as small as 10 nm (ref. 35 ). Finally, owing to the low total condensed mass per air volume (typically 0.1% for a droplet density of 1,000 cm −1 and 1 μm diameter), we neglect the impact of the latent heats of condensation and evaporation on the temperature of the reservoir. How to cite this article: Henin, S. et al . Field measurements suggest the mechanism of laser-assisted water condensation. Nat. Commun. 2:456 doi: 10.1038/ncomms1462 (2011).